STIM1/Orai1 coiled-coil interplay in the regulation of store-operated calcium entry Orai1 calcium channels in the plasma membrane are activated by stromal interaction molecule-1 (STIM1), an endoplasmic reticulum calcium sensor, to mediate store-operated calcium entry (SOCE). The cytosolic region of STIM1 contains a long putative coiled-coil (CC)1 segment and shorter CC2 and CC3 domains. Here we present solution nuclear magnetic resonance structures of a trypsin-resistant CC1–CC2 fragment in the apo and Orai1-bound states. Each CC1–CC2 subunit forms a U-shaped structure that homodimerizes through antiparallel interactions between equivalent α-helices. The CC2:CC2′ helix pair clamps two identical acidic Orai1 C-terminal helices at opposite ends of a hydrophobic/basic STIM–Orai association pocket. STIM1 mutants disrupting CC1:CC1′ interactions attenuate, while variants promoting CC1 stability spontaneously activate Orai1 currents. CC2 mutations cause remarkable variability in Orai1 activation because of a dual function in binding Orai1 and autoinhibiting STIM1 oligomerization via interactions with CC3. We conclude that SOCE is activated through dynamic interplay between STIM1 and Orai1 helices. Store-operated calcium (Ca 2+ ) entry (SOCE) is activated in response to cellular stimuli that deplete the sarco/endoplasmic reticulum (ER) lumen of Ca 2+ , a prerequisite event that opens exquisitely Ca 2+ selective plasma membrane (PM) channels, augmenting cytosolic Ca 2+ levels and refilling ER stores (reviewed in Lewis [1] and Putney [2] ). The principal molecular components of SOCE in many cell types include the ER-inserted stromal interaction molecule-1 (STIM1) [3] , [4] and the Orai1 PM channel subunits [5] , [6] , [7] , [8] , which physically interact at ER–PM junctions in a functional Ca 2+ release-activated Ca 2+ (CRAC) channel complex (reviewed in Muik et al. [9] ). CRAC channels have an extremely high selectivity for Ca 2+ over monovalent ions (that is, >1,000-fold more selective for Ca 2+ than Na + ), a low unitary conductance, a low permeability to large cations (that is, Cs + ) and are regulated by intra- and extracellular Ca 2+ , conferring a unique functional fingerprint among the Ca 2+ channel protein family (reviewed in Prakriya and Lewis [10] ). SOCE through CRAC channels is integral to myriad signalling pathways in electrically excitable and non-excitable cells, the most prominent being immune cells in which inheritable mutations in STIM1 and Orai1 have been linked to devastating immunodeficiency diseases (reviewed in Feske [11] ). Additionally, a role for STIM1 and Orai1 signalling in other pathologies is coming to light such as in breast cancer, for example, where Orai1 expression is upregulated [12] . STIM1 is a type I transmembrane protein with luminal EF-hand and sterile α-motif (SAM) domains that respond to Ca 2+ depletion through intramolecular destabilization of the EF-hand:SAM interface, promoting intermolecular homomerization of this region in SOCE initiation [13] , [14] . The cytosolic architecture of STIM1 is defined by three putative coiled-coil (CC) segments immediately following the single-pass transmembrane (TM) helix and a distal C-terminal Lys-rich region (poly-K) ( Fig. 1a ). STIM1 fragments lacking the luminal and TM domains can activate CRAC entry, independent of Ca 2+ store depletion [15] , [16] , implying that the cytosolic portion is sufficient for eliciting SOCE. Specifically, the Orai-activating STIM fragment (OASF) that includes CC1–CC2–CC3 (that is, residues 233–450/474) encompasses the machinery required for Orai1 activation [17] ; furthermore, the minimal boundaries within OASF required for coupling to and generation of Orai1 currents are found in the CC2–CC3 region. The STIM–Orai-activating region (SOAR) [18] , CRAC-activating domain (CAD) [19] and CC boundary 9 (ref. 20) [20] fragments defined by residues 344–442, 342–448 and 339–446, respectively, can maximally activate Orai1 currents in the absence of store depletion. A CC1–CC2–CC3 (that is, residues 238–462) fragment only activates Orai1 currents after clustering; furthermore, co-clustering of CC1 (that is, residues 238–343) with a spontaneously Orai1-activating CC1–CC2–CC3 fragment (that is, residues 315–462) inhibits Orai1 activity [21] . Hence, while CC2–CC3 contains the minimum domains for Orai1 coupling and activation, the interplay between CC1, CC2 and CC3 modulates the quiescent and activation-competent states of CC2–CC3. Interestingly, a familial R429C mutation in CC3 linked with immunodeficiency and immune dysregulation has a dominant-negative effect on CRAC channel function in patients, without abrogation of full-length protein expression, suggesting a role in STIM1 multimerization and/or STIM1:Orai1 interactions for this CC3 residue position [22] , [23] . 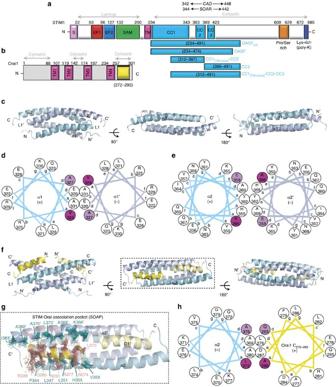Figure 1: NMR structures of apo CC1[TM-distal]-CC2 and the CC1[TM-distal]-CC2:Orai1 C272–292complex. (a) Domain architecture of human STIM1. Amino terminus (N); signal peptide (S); canonical EF-hand (EF1); non-canonical EF-hand (EF2); SAM; TM; putative CC1, CC2 and CC3, respectively; Pro/Ser-rich region; Lys-rich region (poly-K); carboxy terminus (C). Residue ranges are indicated above the domain diagram. Constructs employed in this study are shown below (cyan rectangles) with the residue range (black font) and nomenclature (cyan font) indicated. (b) Domain architecture of human Orai1. Amino terminus (N); TM segments 1, 2, 3 and 4 (TM1, TM2, TM3 and TM4, respectively); carboxy terminus (C). Residue ranges are indicated above the domain diagram. The yellow box delineates the fragment used in this study. (c) Cartoon view of the CC1[TM-distal]-CC2 structure. α1 Helix (α1); loop 1 (L1); α2 helix (α2). Comprehensive structural validation was performed (Supplementary Figs S2c–e, S3 and S4). (d) Supercoiling within the α1:α1′ interface (defg/abcdefg/a=4/7/1). (e) Supercoiling within the α2:α2′ interface (abcdefg/abcd/abcd=7/4/4). (f) Cartoon view of the CC1[TM-distal]-CC2:Orai1 C272–292structure. α1 Helix (α1); Loop 1 (L1); α2 helix (α2); Orai1 C272–292helix (O1). (g) Zoomed view of the SOAP shown inf(broken black boxes). The N-terminal α2 and C-terminal α2′ side chains (sticks) forming one Orai1-binding site are coloured teal. The side chains (sticks) of the Orai1 C272–292peptide, which pack into the pocket, are coloured salmon. (h) Supercoiling within the α2:Orai1 C272–292interface (defg/abcdefg/a=4/7/1). Ind,e,h, the helical wheels show the heptad positions with only reciprocating ‘a’ (purple) and ‘d’ (magenta) packing residues adjacent to one another, not all four residues making up the hole; seeSupplementary Fig. S5a, S5b and S5dfor the proximity and orientation of the ‘a’ and ‘d’ side chains. Figure 1: NMR structures of apo CC1 [TM-distal] -CC2 and the CC1 [TM-distal] -CC2:Orai1 C 272–292 complex. ( a ) Domain architecture of human STIM1. Amino terminus (N); signal peptide (S); canonical EF-hand (EF1); non-canonical EF-hand (EF2); SAM; TM; putative CC1, CC2 and CC3, respectively; Pro/Ser-rich region; Lys-rich region (poly-K); carboxy terminus (C). Residue ranges are indicated above the domain diagram. Constructs employed in this study are shown below (cyan rectangles) with the residue range (black font) and nomenclature (cyan font) indicated. ( b ) Domain architecture of human Orai1. Amino terminus (N); TM segments 1, 2, 3 and 4 (TM1, TM2, TM3 and TM4, respectively); carboxy terminus (C). Residue ranges are indicated above the domain diagram. The yellow box delineates the fragment used in this study. ( c ) Cartoon view of the CC1 [TM-distal] -CC2 structure. α1 Helix (α1); loop 1 (L1); α2 helix (α2). Comprehensive structural validation was performed ( Supplementary Figs S2c–e, S3 and S4 ). ( d ) Supercoiling within the α1:α1′ interface (defg/abcdefg/a=4/7/1). ( e ) Supercoiling within the α2:α2′ interface (abcdefg/abcd/abcd=7/4/4). ( f ) Cartoon view of the CC1 [TM-distal] -CC2:Orai1 C 272–292 structure. α1 Helix (α1); Loop 1 (L1); α2 helix (α2); Orai1 C 272–292 helix (O1). ( g ) Zoomed view of the SOAP shown in f (broken black boxes). The N-terminal α2 and C-terminal α2′ side chains (sticks) forming one Orai1-binding site are coloured teal. The side chains (sticks) of the Orai1 C 272–292 peptide, which pack into the pocket, are coloured salmon. ( h ) Supercoiling within the α2:Orai1 C 272–292 interface (defg/abcdefg/a=4/7/1). In d , e , h , the helical wheels show the heptad positions with only reciprocating ‘a’ (purple) and ‘d’ (magenta) packing residues adjacent to one another, not all four residues making up the hole; see Supplementary Fig. S5a, S5b and S5d for the proximity and orientation of the ‘a’ and ‘d’ side chains. Full size image A high-resolution structure of human SOAR with an L374M/V419A/C437T triple mutation that stabilizes the dimeric state has been solved in the absence of Orai1 (ref. 24) [24] ; however, the structural basis for STIM1:Orai1 interactions, precise CC architecture and conformational changes facilitating Orai1 activation are unresolved. In the present study, we solved the solution nuclear magnetic resonance (NMR) structures of STIM1 CC1–CC2 alone and in complex with the C-terminal domain of Orai1. The structures reveal differences in supercoiling (that is, double α-helix intertwining) in the Orai1-free and -bound states and show that CC2 associates with Orai1 through regions coincidental with the SOAR CC2:CC3 intramolecular interface [24] , suggesting a mode for STIM1 autoinhibition. Further, the orientation of the two human Orai1 C-terminal helices within the CC2:CC2′-created STIM–Orai association pocket (SOAP) is highly analogous with the Drosophila C-terminal helices in the dimer units of the crystallized Orai hexamer [25] , suggesting a mechanism of STIM1:Orai1 C-terminus coupling in the CRAC complex assembly. STIM1 CC1 [TM-distal] -CC2 structure Limited tryptic digestion was used to identify compact domains within the larger cytosolic OASF/OASF ext fragments, revealing two major proteolysis-resistant fragments: a segment overlapping CC1 and CC2 (that is, residues 312–387, renamed CC1 [TM-distal] -CC2) and a second region consisting of CC3 alone (that is, residues 388–474/491, renamed CC3) ( Supplementary Table S1 ; Supplementary Fig. S1a,b ; Supplementary Discussion ). Lengthening the CC1 [TM-distal] -CC2 core to include CC3 enhanced the protein stability and dimerization, more comparable to OASF ext ( Supplementary Fig. S1c–h ). However, the CC1 [TM-distal] -CC2 protein proved to be the most amenable one for solution NMR studies following buffer optimization ( Supplementary Fig. S2a,b ; Supplementary Discussion ). The solution structure of CC1 [TM-distal] -CC2 was solved using an Nuclear Overhauser effect (NOE)-derived distance-based approach ( Table 1 ). The structure of CC1 [TM-distal] -CC2 exhibits two extended helices (that is, α1, residues 313–340; α2, residues 344–382) linked through a short loop (that is, L1, residues 341–343) and arranged in an antiparallel manner ( Fig. 1c ). Two U-shaped monomers form an antiparallel and symmetric dimer through α1:α1′, α2:α2′ and C-terminal α2:L1′ contacts ( Fig. 1c ). Since low levels of 2,2,2-trifluoroethanol (TFE) were required to produce homogeneous NMR spectra, we used far-UV circular dichroism (CD), small angle X-ray scattering (SAXS) and dynamic light scattering (DLS) in the absence of TFE to validate the CC1 [TM-distal] -CC2 structure ( Supplementary Figs S2c–e,S3 and S4 ; Supplementary Table S2 ; Supplementary Discussion ); however, it is possible that the low resolution and species-averaging information reported by these techniques could mask conformational effects of TFE only detectable using high-resolution methods (that is, NMR and X-ray crystallography). Hence, we used extensive structure-rationalized and site-specific mutagenesis in combination with far-UV-CD, size exclusion chromatography (SEC) with in-line multi-angle light scattering, pull-down experiments, live-cell electrophysiology and fluorescent colocalization studies in the absence of TFE to further substantiate our high-resolution structures and the structure-derived functional models. Table 1 NMR statistics for the apo CC1 [TM-distal] -CC2 structure ensemble. Full size table We used SOCKET [26] to locate the CC interaction network and heptad positions within the CC1 [TM-distal] -CC2 structure. Consistent with primary sequence prediction, two key CC interactions were recognized. One symmetric antiparallel CC forms along residues E320 to A331 of each subunit with V324 and A327 side chains occupying the buried ‘a’ and ‘d’ knob positions in a canonical heptad repeat, respectively, that pack into holes made up of four residues that include reciprocating ‘a’ and ‘d’ knobs from the partner helix ( Fig. 1d ). More extensive left-handed supercoiling is observed in the second symmetric antiparallel CC along α2 residues H355 to A369; the α2 CC exhibits one discontinuity in the heptad repeat with E358 and K366 occupying the critical ‘a’ and ‘d’ positions, respectively ( Fig. 1e ). The Y342 and A343 residues of L1 are positioned to interact with the C-terminal end of the α2′ helix, and although A376′, A380′ and I383′ residues are in close proximity to L1 ( Supplementary Fig. S5c ), the L1:α2′ contacts appear only marginally stable as the α2 C-terminal region shows high internal dynamics ( Supplementary Fig. S6 ). Consistent with the increased structural variability (that is, relatively higher backbone root mean square deviation (rmsd)) at the N- and C-termini of the ensemble (Supplementary Fig. S6a), 15 N-{ 1 H} heteronuclear NOE measurements show decreased saturated/reference peak intensity ratios, indicating greater mobility on the ~ns timescales compared with the central α1 and α2 regions, which exhibit the highest ratios (Supplementary Fig. S6b,c). The most rigid backbone regions within apo CC1 [TM-distal] -CC2 are congruent with the α1:α1′ and α2:α2′ CC configurations observed in dimer stabilization. The increased dynamics at the termini reflect regions of conformational instability that are apt to undergo or initiate structural changes related to regulatory mechanisms. STIM1 CC1 [TM-distal] -CC2:Orai1 C 272–292 complex structure STIM1 binding to both the Orai1 N- and C-terminal domains are required for recruitment and gating at ER–PM junctions; however, the interaction with the Orai1 C-terminal domain occurs with higher apparent affinity than the N-terminal domain, as deletion of the N-terminal domain completely abolishes channel activity but not the ability to co-cluster with STIM1, whereas deletion of the C-terminal domain eliminates the interaction [9] , [16] , [19] , [27] , [28] , [29] . We engineered a glutathione- S -transferase (GST)-Orai1 C 272–292 fusion (that is, Orai1 residues 272–292) ( Fig. 1b ), which exhibited resistance to degradation and was soluble to >3 mM after GST cleavage. NMR chemical-shift perturbation data demonstrated Orai1 C 272–292 binding to STIM1 CC1 [TM-distal] -CC2. Specifically, the CC1 [TM-distal] -CC2 1 H- 15 N-HSQC (heteronuclear single quantum coherence) spectrum exhibited residue-specific chemical-shift perturbations upon addition of unlabelled Orai1 C 272–292 up to 2 mM ( Supplementary Fig. S7a ). Similarly, we observed chemical-shift changes in a titration of unlabelled CC1 [TM-distal] -CC2 into uniformly 15 N-Orai1 C 272–292 ( Supplementary Fig. S7b ). The NMR spectra of the mixed samples exhibited no peak doubling, indicating that this dimeric STIM1 fragment maintains two equivalent Orai1 C 272–292 -binding sites with single magnetic environments at all residue positions. The greatest chemical-shift changes observed in the Orai1 C 272–292 1 H- 15 N-HSQC spectrum occurred on both the N- and C-terminal halves of the peptide and included residues E272, L273, N274, A277, E278, A280, R281, H288 and R289 ( Supplementary Fig. S7c ). The ability of CC1 [TM-distal] -CC2 to bind Orai1 C 272–292 in the absence of TFE was confirmed using pull-down experiments ( Supplementary Fig. S7d ; Supplementary Discussion ). We used the perturbation data to estimate the concentration of protein or peptide required to saturate our NMR samples ( Supplementary Fig. 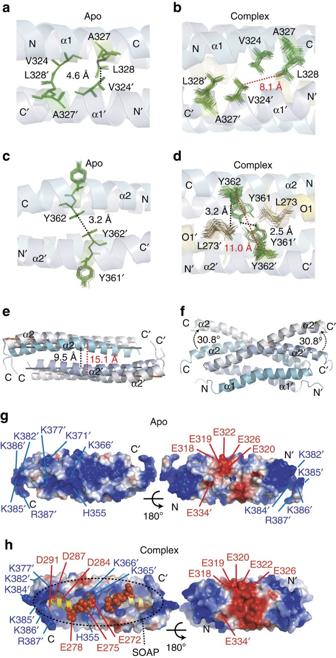Figure 2: CC1[TM-distal]-CC2 structural changes associated with Orai1 C272–292binding. (a) V324 and L328′ side-chain (green sticks) proximity in the apo α1:α1′ interface. The distance between the V324-Cβand L328′-Cγatoms is indicated (broken black line). (b) V324 and L328′ side-chain (green sticks) proximity in the α1:α1′ interface of the CC1[TM-distal]-CC2:Orai1 C272–292structure. The distance between the V324-Cβand L328′-Cγatoms is indicated (red broken line). (c) Central pivot point of the apo α2:α2′ interface. The intermolecular Y362-OH (green sticks) distance (broken black line) is shown. (d) Central α2:α2′ pivot point in the CC1[TM-distal]-CC2:Orai1 C272–292structure. The intermolecular Y362-OH (green sticks) distance (broken red line) is shown. The Orai1 L273-Cγ(brown sticks) to Y362-OH and intermolecular Y361-OH (green sticks) distances (broken black lines) are also shown. (e) Distance between the α2 helical axes in the apo (blue cartoons; broken black line) versus Orai1 C272–292-bound (white cartoons; broken red line) states. (f) Angular opening (broken curved line) of the C-terminal α2 region upon Orai1 C272–292binding. The apo α2 helices (blue cartoons) are shown relative to Orai1-bound α2 helices (white cartoons). (g) Surface electrostatics of the CC1[TM-distal]-CC2 structure. The distinct α1:α1′ acidic and the C-terminal basic residues are labelled. (h) Electrostatic complementarity between CC1[TM-distal]-CC2 and Orai1 C272–292derived from the complex structure. The basic rim residues of the SOAP (broken black circle) and acidic patches are labelled. The Orai1 C272–292peptides (yellow cartoons) and the acidic side chains are shown (red space fill). The electrostatic gradient ing,his from −2 (red) to +2 (blue) kT/e. S7e ) and proceeded to determine the solution structure of STIM1 CC1 [TM-distal] -CC2 in complex with Orai1 C 272–292 using NOE-derived distance restraints ( Table 2 ). The dimeric STIM1 protein equivalently binds two Orai1 C 272–292 molecules ( Fig. 1f ); furthermore, the Orai1 C 272–292 -binding pocket (that is, SOAP) within the STIM1 CC1 [TM-distal] -CC2 region is formed primarily by side chains of the α2 helices; specifically, P344, L347, L351, H355 and V359 from the N-terminal side of α2 on one subunit and Y362′, K366′, A369′, L373′, A376′, A380′ and I383′ from the C-terminal side of α2′ on the second subunit form a predominantly hydrophobic groove that accommodates one Orai1 C 272–292 molecule ( Fig. 1g ). Side chains from two sides of one Orai1 α-helix pack against opposite faces of the SOAP. The N274, A277, R281, Q285 and R289 Orai1 residues interact with the N-terminal α2 surface, while L273, L276, A280, Q283 and L286 residues interact with the C-terminal side of the second α2′ subunit within the SOAP ( Fig. 1g ). Table 2 NMR statistics for the CC1 [TM-distal] -CC2:Orai1 C 272–292 complex structure. Full size table Analysis of the complex structure using SOCKET [26] revealed the absence of supercoiling at the α1:α1′ and α2:α2′ interfaces. Instead, two new parallel CC interactions are formed along L276 to D287 within each Orai1 C 272–292 domain and residues A369 to A380 within each of the STIM1 α2 helices ( Fig. 1h ). The ‘a’ and ‘d’ positions of the α2 helices are occupied by L373 and A376, respectively, while A280 and Q283 residues of Orai1 are in the ‘a’ and ‘d’ positions, respectively ( Fig. 1h ). The supercoiling occurs through uninterrupted heptad repeats in 12 residue stretches of the STIM1 α2 and Orai1 C-terminal helices. STIM1 conformational changes upon Orai1 C 272–292 binding Along with the ‘a’ and ‘d’ interactions, the α1:α1′ interface exhibits central V324:L328′ hydrophobic side-chain packing in the absence of Orai1 C 272–292 binding ( Fig. 2a ). In complex with Orai1 C 272–292 , the α1 helices undergo a registry shift, facilitating closer V324:V324′ side-chain interactions. The helix registry shift causes the distance between the V324-C β and L328′-C γ atoms to increase from ~4.6 Å in the apo state to ~8.1 Å in the Orai1 C 272–292 -bound state ( Fig. 2b ). Two marked conformational changes occur in the α2:α2′ interface to accommodate the Orai1 C 272–292 peptides at opposite ends of the SOAP. First, the α2 helices become separated in the Orai1 C 272–292 -bound state compared with the apo state. This α2:α2′ dilation is illustrated by the Y362:Y362′ pivot point residues, which move from a distance of ~3.2 Å in the apo form ( Fig. 2c ) to ~11.0 Å in the Orai1 C 272–292 -bound state (OH groups; Fig. 2d ); moreover, the distance between the α2 helical axes increases by ~5.6 Å after this separation ( Fig. 2e ), and the Y362 side chains interact with L273 of the Orai1 C 272–292 peptides ( Fig. 2d ). Second, the C-terminal half of the α2 helices hinge away from L1′ by ~30.8° at the Y362 pivot point ( Fig. 2f ). This angular opening of the α2 helices allows supercoiling with Orai1 C 272–292 in the SOAP to occur. Figure 2: CC1 [TM-distal] -CC2 structural changes associated with Orai1 C 272–292 binding. ( a ) V324 and L328′ side-chain (green sticks) proximity in the apo α1:α1′ interface. The distance between the V324-C β and L328′-C γ atoms is indicated (broken black line). ( b ) V324 and L328′ side-chain (green sticks) proximity in the α1:α1′ interface of the CC1 [TM-distal] -CC2:Orai1 C 272–292 structure. The distance between the V324-C β and L328′-C γ atoms is indicated (red broken line). ( c ) Central pivot point of the apo α2:α2′ interface. The intermolecular Y362-OH (green sticks) distance (broken black line) is shown. ( d ) Central α2:α2′ pivot point in the CC1 [TM-distal] -CC2:Orai1 C 272–292 structure. The intermolecular Y362-OH (green sticks) distance (broken red line) is shown. The Orai1 L273-C γ (brown sticks) to Y362-OH and intermolecular Y361-OH (green sticks) distances (broken black lines) are also shown. ( e ) Distance between the α2 helical axes in the apo (blue cartoons; broken black line) versus Orai1 C 272–292 -bound (white cartoons; broken red line) states. ( f ) Angular opening (broken curved line) of the C-terminal α2 region upon Orai1 C 272–292 binding. The apo α2 helices (blue cartoons) are shown relative to Orai1-bound α2 helices (white cartoons). ( g ) Surface electrostatics of the CC1 [TM-distal] -CC2 structure. The distinct α1:α1′ acidic and the C-terminal basic residues are labelled. ( h ) Electrostatic complementarity between CC1 [TM-distal] -CC2 and Orai1 C 272–292 derived from the complex structure. The basic rim residues of the SOAP (broken black circle) and acidic patches are labelled. The Orai1 C 272–292 peptides (yellow cartoons) and the acidic side chains are shown (red space fill). The electrostatic gradient in g , h is from −2 (red) to +2 (blue) kT/e. Full size image The surface of apo CC1 [TM-distal] -CC2 structure is markedly basic in amino-acid composition; however, the α1:α1′ supercoiling facilitates the formation of a negative patch by orienting E318, E319, E320 and E322 residues of the two subunits close to one another ( Fig. 2g ). This acidic region is not interfacial with the α2 C-terminal basic stretch of amino acids (that is, K382, K384, K385, K386 and R387) previously suggested to keep STIM1 in a quiescent state through an electrostatic clamp [21] ; however, longer-range charge attractions between these structural features may help position the α2 C-terminal region close to L1′. The acidic stretch of residues on each α1 helix (that is, E318, E319, E320 and E322) is closer to the identical stretch on the second subunit in the Orai1 C 272–292 -bound versus the apo state, creating a large contiguous negative patch on the α1:α1′ face ( Fig. 2h ). The surface of the SOAP is primarily positive created by H355, K365′, K366′, K377′, K382′, K384′, K385′, K386′ and R387′ of the α2 helices ( Fig. 2h ). This SOAP basicity is complementary to the predominantly negative surface of each Orai1 C 272–292 helix created by acidic residues including E272, E275, E278, D284, D287 and D291 and likely contributes to the stability of the complex ( Fig. 2h ). Several aspects of the CC1 [TM-distal] -CC2 dimer backbone dynamics are consistent with the structural changes accompanying the binding of two Orai1 C 272–292 peptides in an antiparallel manner ( Supplementary Fig. S8a ). First, the increased variability in the 15 N-{ 1 H} NOE ratios compared with the apo state can be attributed to relatively weak peptide binding, promoting conformational exchange ( Supplementary Fig. S8b ). Second, the decrease in the backbone dynamics of the N-terminal region (that is, residues 312–316) is consistent with the registry shift moving the α1:α1′ interaction site closer to the termini, thereby decreasing mobility of the termini ( Supplementary Fig. S8b ). Most importantly, the attenuated backbone mobility compared with the apo state, observed at the N- and C-terminal regions of α2 that create the SOAP, correlates with the Orai1 C 272–292 -binding sites ( Supplementary Fig. S8b,c ). STIM1 CC1 [TM-distal] -CC2 structural integrity in SOCE What is the correlation between CC1 [TM-distal] -CC2 structural integrity and the ability of STIM1 to activate Orai1 channels? We answered this question using patch-clamp electrophysiology experiments of HEK-293 cells co-overexpressing full-length monomeric Cherry fluorescent protein (mCh)-STIM1 and YFP-Orai1 ( Fig. 3a ) after in vitro assessments of the affect of mutations ( Supplementary Fig. S9a ) on the folding, stability and dimerization propensity of CC1 [TM-distal] -CC2 ( Supplementary Table S3 ; Supplementary Discussion ). Cells co-overexpressing the STIM1 E318Q/E319Q/E320Q/E322Q (that is, 4EQ) charge-neutralizing quadruple mutant, which stabilized the α1:α1′ interface and promoted dimerization of the CC [TM-distal] -CC2 region ( Supplementary Figs S1h,S10a and S11a ), exhibited spontaneous inward-rectifying currents at the time of patch pipette break-in ( Fig. 3b,i ). The inward currents were blocked by La 3+ , confirming a CRAC channel-dependent entry. Disruption of the α1:α1′ interaction and destabilization of the CC1 [TM-distal] -CC2 dimer via the V324P mutation ( Supplementary Figs S1h,S10b and S11b ) significantly attenuated the maximal inward-rectifying current compared with the wild type after passive ER Ca 2+ store depletion with EGTA ( Fig. 3c,i ), underscoring the importance of an intact α1:α1′ interface to transduce a conformation that maximally activates CRAC entry. These data suggest that the α1 structural integrity plays an important role in the quiescent-to-active STIM1 transduction efficiency; furthermore, the meta-stability of α1 conferred by the acidic cluster ensures that the region is readily susceptible to allosteric changes. Consistent with this notion, the 4EQ mutant that increased the CC1 [TM-distal] -CC2 dimer propensity enhanced the CC1 [TM-distal] -CC2 interaction with Orai1 C 272–292 , while the V324P mutation that disrupted CC1 [TM-distal] -CC2 dimerization diminished the CC1 [TM-distal] -CC2:Orai1 C 272–292 interaction ( Supplementary Fig. S7d ). 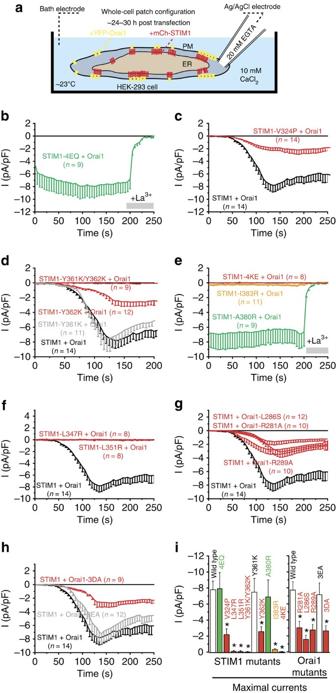Figure 3: Affects of CC1[TM-distal]-CC2:Orai1 C272–292mutations on full-length function. (a) Whole HEK-293 cell patch-clamp configuration used in this study. Current densities were measured at −86 mV. (b–f) Inward-current plots of cells co-overexpressing wild-type YFP-Orai1 and full-length mCh-STIM1 4EQ (b), V324P (c), Y361K/Y362K, Y362K or Y361K (d), A380R, I383R or 4KE (e) and L347R or L351R (f). (g,h) Inward-current plots of cells co-overexpressing wild-type mCh-STIM1 and mutant YFP-Orai1 R281A, L286S or R289A (g) and D284A/D287A/D291A or E272A/E275A/E278A (h). (i) Summary graph of maximal inward currents. Green bars represent spontaneous maximally activated currents and red bars indicate significantly attenuated maximal currents. The Orange bar represents I383R, which showed spontaneous inward currents slightly above background. Data are means±s.e.m. forn, number of cells and asterisks denote *P<0.05 by two-tailed Student’st-test. Curve colours match the residues inSupplementary Fig. S9a,b. SeeSupplementary Table S3forin vitro(Supplementary Figs S10 and S11) and live-cell data summary. Figure 3: Affects of CC1 [TM-distal] -CC2:Orai1 C 272–292 mutations on full-length function. ( a ) Whole HEK-293 cell patch-clamp configuration used in this study. Current densities were measured at −86 mV. ( b – f ) Inward-current plots of cells co-overexpressing wild-type YFP-Orai1 and full-length mCh-STIM1 4EQ ( b ), V324P ( c ), Y361K/Y362K, Y362K or Y361K ( d ), A380R, I383R or 4KE ( e ) and L347R or L351R ( f ). ( g , h ) Inward-current plots of cells co-overexpressing wild-type mCh-STIM1 and mutant YFP-Orai1 R281A, L286S or R289A ( g ) and D284A/D287A/D291A or E272A/E275A/E278A ( h ). ( i ) Summary graph of maximal inward currents. Green bars represent spontaneous maximally activated currents and red bars indicate significantly attenuated maximal currents. The Orange bar represents I383R, which showed spontaneous inward currents slightly above background. Data are means±s.e.m. for n , number of cells and asterisks denote * P <0.05 by two-tailed Student’s t -test. Curve colours match the residues in Supplementary Fig. S9a,b . See Supplementary Table S3 for in vitro ( Supplementary Figs S10 and S11 ) and live-cell data summary. Full size image Our structures revealed centrally located, double Tyr residues within the α2 helices; hence, the Y361K/Y362K double Tyr mutation was engineered to fully eliminate the thermodynamically favourable propensity for Tyr-Tyr stacking [30] , [31] at this central α2:α2′ crossover point. The Y361K/Y362K double mutation completely precluded the ability of full-length STIM1 to activate CRAC entry ( Fig. 3d,i ), consistent with disruption of the α2:α2′ interface and CC1 [TM-distal] -CC2 dimer destabilization ( Supplementary Figs S1h,S10c and S11c ). Further, the Y361K/Y362K double mutation suppressed CC1 [TM-distal] -CC2 binding to Orai1 C 272–292 ( Supplementary Fig. S7d ). While inhibition of the SOAP formation was a principal cause of this phenotype, Y362′ interacts with Orai1 L273, also suggesting that the perturbation of intermolecular side-chain packing may have been involved. Consistent with this notion, a single Y362K substitution within STIM1 significantly reduced maximal currents upon store depletion compared with the wild type ( Fig. 3d,i ). These data demonstrate that an intact α2:α2′ interaction is necessary to induce an activation-competent STIM1 conformation. The possibility that the Y361K/Y362K double mutant causes gross unfolding of the resting SOAR dimer cannot be discounted. Additionally, the Y361K mutation could potentially disrupt contacts with α1′; however, since STIM1-Y361K is capable of eliciting maximal Orai1 currents ( Fig. 3d,i ), this scenario is unlikely. Our NMR structures revealed that the C-terminal region of α2 hinges away from L1′ by >30° upon Orai1 C 272–292 binding compared with the apo state ( Fig. 2f ). Interestingly, C-terminal α2 mutations that may affect CC2 homomerization as well as heteromerization with the Orai1 C-terminal domain produce somewhat disparate CRAC current profiles. Cells co-overexpressing Orai1 and STIM1 A380R show constitutive CRAC entry characterized by maximal inward-current density at the time of break-in and La 3+ inhibition ( Fig. 3e,i ). STIM1 I383R induces Orai1 currents only slightly above the background but is inhibited by La 3+ ( Fig. 3e,i ). The preservation of the CC1 [TM-distal] -CC2:Orai1 C 272–292 interaction observed with the A380R and I383R mutants ( Supplementary Fig. S7d ) is congruent particularly with the A380R-induced constitutive CRAC activation, and since both the mutations only marginally affect the stability, folding and dimer propensity of CC1 [TM-distal] -CC2 ( Supplementary Figs S1h,S10d,e and S11d,e ), these residues must be involved in other aspects of the signalling process, such as an intramolecular transition in STIM1 prerequisite to adopting an Orai1 activation-competent state [21] , [32] and/or Orai1 N-terminal interactions. It should be noted that A380 and I383 residues are relatively distant (that is, ~20–25 Å) from the Orai N-terminus in our assembled channel-coupling model (see below); however, additional high-resolution data are required to completely rule out interactions with the Orai1 N-terminus. Disruption of the surface basicity at the C-terminal α2 region via the K382E/K384E/K385E/K386E (that is, 4KE) quadruple mutation, which only marginally alters the stability, folding and dimerization of CC1 [TM-distal] -CC2 compared with the wild type ( Supplementary Figs S1h,S10f and S11f ), completely abrogates CC1 [TM-distal] -CC2:Orai1 C 272–292 interactions ( Supplementary Fig. S7d ) as well as inward CRAC current ( Fig. 3e,i ), advocating a role for electrostatic complementarity in STIM1:Orai1 coupling and the activation of CRAC entry. Taken together, these data demonstrate that the α2:L1′ interface minimally affects the CC1 [TM-distal] -CC2 dimer structure, consistent with the high backbone mobility of the C-terminal α2 region ( Supplementary Fig. S6 ); however, residues of the C-terminal α2 region are involved in multiple facets of CRAC channel activation, including coupling to Orai1 and aspects currently unresolved in available high-resolution structures ( Supplementary Discussion ). STIM1 CC1 [TM-distal] -CC2:Orai1 C 272–292 interface in SOCE We employed live-cell patch-clamp experiments in conjunction with rationalized mutagenesis ( Supplementary Fig. S9b ) to validate the structurally elucidated STIM1:Orai1 interactions. First, we separately introduced L347R and L351R mutations into full-length STIM1, aimed at disrupting the N-terminal α2 hydrophobic face of the SOAP, while maintaining the electrostatic complementarity to Orai1. Cells co-overexpressing Orai1 and STIM1 with these substitutions exhibited no inward-rectifying current upon passive Ca 2+ store depletion ( Fig. 3f,i ); furthermore, OASF-L347R and -L351R mutants had no ability to colocalize with Orai1 at the PM ( Supplementary Fig. S9c,d ). We separately engineered R281A, L286S and R289A mutations in full-length Orai1, as these amino acids were identified to make contacts within the SOAP and have not been previously studied ( Supplementary Discussion ). Co-overexpression of each of these full-length Orai1 mutants with wild-type STIM1 resulted in significantly attenuated maximal Orai1 currents after store depletion ( Fig. 3g,i ). Three anionic Glu amino acids (that is, E272, E275 and E278) are located on the N-terminal half and three Asp residues (that is, D284, D287 and D291) are present on the C-terminal half of Orai1 C 272–292 . Cells co-overexpressing an Orai1 E272A/E275A/E278A triple mutant with wild-type STIM1 did not appreciably affect the current–density profiles compared with the wild-type Orai1 ( Fig. 3h,i ). However, the Orai1 D284A/D287A/D291A triple mutant significantly attenuated the maximum inward currents versus wild type ( Fig. 3h,i ). Hence, the acidic D284, D287, D291 triplet within Orai1 C 272–292 plays a dominant role in complementing the electropositive surface of the SOAP and is consistent with a close proximity to the basic C-terminal α2 stretch (that is, K382′, K384′, K385′ and K386′) elucidated in the complex structure. All Orai1 mutations that inhibited CRAC currents also attenuated colocalization with STIM1-OASF at the PM ( Supplementary Fig. S9c,e ), suggesting reduced STIM1:Orai1 coupling. Hence, both non-polar and polar forces promote Orai1 C 272–292 binding to CC1 [TM-distal] -CC2. The present structures of apo and Orai1 C 272–292 -complexed STIM1 CC1 [TM-distal] -CC2 complemented by in vitro biophysical and live-cell functional analyses have illuminated several mechanistic features of STIM1-Orai1 signalling. First, the nature of the CC1:CC1′ interaction is coupled to the efficiency of Orai1 activation by STIM1. CC1 [TM-distal] :CC1 [TM-distal] ′ interactions that favour a dimer conformation promote coupling to and activation of Orai1, as evidenced by the 4EQ mutant, which increases dimer propensity and stability of CC1 [TM-distal] -CC2, resulting in constitutive Orai1 currents in the full-length STIM1 context ( Supplementary Table S3 ). A STIM1 E318A/E319A/E320A/E322A (that is, 4EA) mutant, previously shown to constitutively activate CRAC channels in Orai1 co-overexpressing COS-7 cells [21] , likely has a similar mode of action as 4EQ. Of the 4E residues in the 4EQ and 4EA mutants (that is, E318, E319, E320 and E322), only E322 (that is, E264 in Caenorhabditis elegans ) contacts the CAD/SOAR region based on the C. elegans STIM crystal structure (3TER.pdb); furthermore, deletion of residues 318–322 containing the 4E stretch does not alter the Ca 2+ store-dependent wild-type behaviour of STIM1 in terms of puncta formation and Orai1 activation [33] . Taken together, these data suggest that the mechanism by which the 4EQ and 4EA mutations constitutively activate Orai1 is distinct from the effects of the 310–337 deletion mutant [24] , which probably eliminates all folding constraints on the CAD/SOAR region, resulting in constitutively Orai1 activation. Disruption of CC1 [TM-distal] via a helix-breaking V324P mutation destabilizes CC1 [TM-distal] -CC2 and promotes monomer, resulting in less efficient Orai1 activation ( Supplementary Table S3 ; Supplementary Discussion ). Second, each STIM1 dimer forms two identical Orai1 C 272–292 -binding sites through an antiparallel configuration of the α2 helices, positioning N- and C-terminal α2 residues on opposite faces of each binding site within the SOAP ( Fig. 1g ). All previously identified STIM1 cytosolic fragments, which activate Orai channels preserve the SOAP (that is, CAD [19] , SOAR [18] , OASF [17] and CC boundary 9 (ref. 20) [20] ). This structural organization is corroborated by several previous studies demonstrating that the efficacy of CRAC channel activation by CAD/SOAR in live cells is sensitive to truncations and mutations at the N-terminus of α2. For example, the L347A/Q348A mutation abolishes SOAR colocalization and co-immunoprecipitation with Orai1 (refs 18 , 24 ). Moreover, L273S and L276D mutations in the Orai1 C-terminal domain strongly inhibit CRAC entry [16] , [18] , [34] , and our data reveal that these non-polar residues contact opposite sides within one hydrophobic cleft of the SOAP ( Fig. 1g ). Further, STIM1 fragments that exclude ~6–8 residues from the N-terminal α2 helix (that is, fragments encompassing residues 350–450 or 350–448) inefficiently induce CRAC entry compared with CAD and SOAR fragments, which retain these residues [18] , [19] . Mutations on the α2 C-terminal face of the SOAP can also disrupt Orai1 activation. The OASF L373S mutant fails to induce constitutive Orai1 currents concomitant with a decrease in STIM1:Orai1 colocalization [27] . STIM1 A376K constitutively forms puncta at resting ER Ca 2+ , with no ability to recruit Orai1 to these ER–PM sites [35] . The non-polar interactions within the SOAP are reinforced by charge complementarity (that is, STIM1 K382, K384, K385, K386 with Orai1 D284, D287, D291), an interaction mechanism first proposed by Baird and co-workers [36] , [37] who showed that K384Q/K385Q/K386Q or Orai1 E272Q/E275Q/E278Q/D284N/D287N/D291N mutations can abolish STIM1:Orai1 colocalization and SOCE. Foremost, our structural data reveal that the supercoiling changes from the apo CC1 [TM-distal] -CC2 to the Orai1 C 272–292 -complexed state, suggesting a dynamic CC interplay is involved in the activation of Orai1 channels. In the apo STIM1 state, CC1 [TM-distal] -CC2 exhibits intersubunit (that is, α1:α1′ and α2:α2′) CC interactions, constricting the SOAP within the α2 CC interface. Complexed with Orai1 C 272–292 , the homotypic intersubunit supercoiling is alleviated and, instead, STIM1 engages in heterotypic α2:Orai1 C 272–292 supercoiling. Structural alignment of CC2 from the SOAR structure [24] with CC2 of the apo CC1 [TM-distal] -CC2 and CC1 [TM-distal] -CC2:Orai1 C 272–292 structures shows that CC3 of SOAR occupies the same position as CC2′ (that is, a2′) of the apo structure ( Supplementary Fig. S12a ) and Orai1 C 272–292 within the complex structure ( Supplementary Fig. S12b ). The analogous positions allude to an elegant CC-switching mechanism involved in CRAC activation (see below). The STIM1 CC3 region drives the oligomerization of the cytosolic domains necessary to activate Orai1 channels, as previous work showed that STIM1 residues 420–450 are required for the enhancement of STIM1 homomerization as well as CRAC activation [17] , and residues 392–448 are essential for stabilizing higher-order STIM1 oligomers after ER Ca 2+ store depletion [35] . Indispensible CC3-mediated oligomerization is also congruent with reports showing that C-terminal truncations decrease the intermolecular FRET between CAD molecules [35] and markedly disrupt the ability of SOAR fragments to activate Orai1 (ref. 18) [18] . We speculate that the SOAR crystalline state represents a quiescent, non-Orai1-coupled structure, which may undergo a conformational change such that the CC2:CC2′ orientation mimics that observed in the apo CC1 [TM-distal] -CC2 solution structure prior to coupling with and gating of the Orai channels. The basis for this speculation includes the facts that SOAR CC2:CC3 interface mutations can cause an OASF extension, which has been linked with Orai1 activation [32] , and the apo CC1 [TM-distal] -CC2 structure is more analogous to the Orai1 C 272–292 -complexed state and appears better primed for the Orai1 C-terminal interaction. Recently, Drosophila melanogaster Orai was crystallized in a hexameric conformation with individual dimers stabilized through antiparallel CC interactions between the cytosolic C-terminal helices [25] . Remarkably, the antiparallel configuration of the Orai C-terminal helices in D. melanogaster appears primed for an interaction with STIM, highly analogous to the one elucidated in our human STIM1 CC1 [TM-distal] -CC2:Orai1 C 272–292 complex structure ( Fig. 4a ). The interhelix angle between the two interacting D. melanogaster Orai C-terminal helices (that is, 152°) is very similar to the angle observed in our human complex structure (that is, 136°) ( Fig. 4a ). Docking of three dimer structures of CC1 [TM-distal] -CC2:Orai1 C 272–292 on the Orai hexamer by structurally aligning the common Orai C-terminal regions ( Fig. 4b,c ) confirms the noteworthy structural compatibility. Specifically, the N-termini of CC1 [TM-distal] -CC2, indicating the positions of CC1 [TM-proximal] , are directed away from the cytosolic channel face towards the ER membrane; further, the C-termini of CC1 [TM-distal] -CC2, marking the locations of CC3, are adjacent to the C-termini from neighbouring CC1 [TM-distal] -CC2 dimers and are compatible with homotypic oligomerization of CC1 [TM-distal] -CC2 via CC3 interactions into a required functional stoichiometry ( Fig. 4b ). 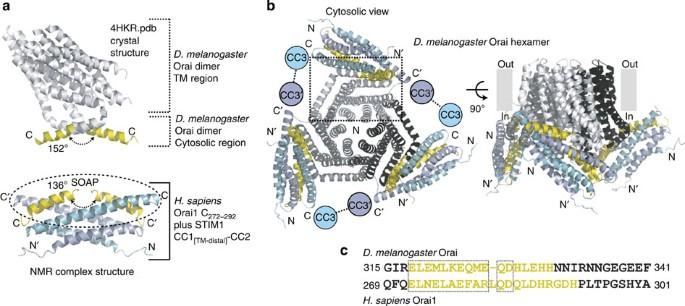Figure 4: Docking of CC1[TM-distal]-CC2 on the Orai hexamer. (a) Structural homology betweenD. melanogasterOrai and human Orai1 C272–292. TheD. melanogasterOrai dimer (top) shows an antiparallel C-terminal configuration (yellow) highly homologous to human Orai1 C272–292(bottom; yellow). The analogous interhelix angles indicated (broken curved lines). (b) Docking of CC1[TM-distal]-CC2 onto hexamericD. melanogasterOrai. The Orai1 C272–292helices within the CC1[TM-distal]-CC2 complex were structurally aligned through sequentially similar regions in eachD. melanogasterOrai dimer. CC3 locations are inferred from the position of the α2 C-termini. The Orai dimer unit is indicated (broken black box). (c) Sequence alignment ofD. melanogasterOrai andH. sapiensOrai1 C-terminal residues. TheH. sapiensOrai1 C272–292residues and the homologous residues visible in theD. melanogastercrystal structure are yellow. The boxed residues indicate the structurally aligned regions. Figure 4: Docking of CC1 [TM-distal] -CC2 on the Orai hexamer. ( a ) Structural homology between D. melanogaster Orai and human Orai1 C 272–292 . The D. melanogaster Orai dimer (top) shows an antiparallel C-terminal configuration (yellow) highly homologous to human Orai1 C 272–292 (bottom; yellow). The analogous interhelix angles indicated (broken curved lines). ( b ) Docking of CC1 [TM-distal] -CC2 onto hexameric D. melanogaster Orai. The Orai1 C 272–292 helices within the CC1 [TM-distal] -CC2 complex were structurally aligned through sequentially similar regions in each D. melanogaster Orai dimer. CC3 locations are inferred from the position of the α2 C-termini. The Orai dimer unit is indicated (broken black box). ( c ) Sequence alignment of D. melanogaster Orai and H. sapiens Orai1 C-terminal residues. The H. sapiens Orai1 C 272–292 residues and the homologous residues visible in the D. melanogaster crystal structure are yellow. The boxed residues indicate the structurally aligned regions. Full size image Our solution NMR structures and functional data in conjunction with recent CRAC component crystal structures convey a CC-switching mechanism in the transition of the cytosolic STIM1 region from a quiescent to an Orai1 activation-competent state. We propose that intramolecular CC2:CC3 supercoiling ( Supplementary Fig. S12c ; Supplementary Discussion ) contributes to the suppression of CC3-mediated STIM1 assembly and internal autoinhibition of intermolecular CC2:CC2′ as well as CC2:Orai1 C 272–292 interactions, since CC3 occupies the same space as CC2′ and Orai1 C 272–292 after structural alignment of CC2 ( Fig. 5a ; Supplementary Fig. S12a,b ). Store depletion drives self-association of CC1 [TM-proximal] , which induces a cytosolic domain rearrangement [32] , [38] that we believe favours the α1:α1′ CC interaction elucidated in our apo structure. Accessing this conformation releases the intramolecular CC2:CC3 supercoiling, permitting the structurally elucidated intermolecular CC2:CC2′ supercoiling ( Fig. 5a ). Critically, the antiparallel α2:α2′arrangement forms the SOAP, which ultimately facilitates α2:Orai1 C 272–292 supercoiling upon complexation. The released CC3 module promotes the assembly of STIM1 dimers into higher-order oligomers such as hexamers ( Fig. 5b ) or tetramers ( Supplementary Fig. S13a ) through CC3:CC3′ interactions. Recent studies show that concatenated hexameric Orai1 is permeable to Na + and Cs + ions in addition to Ca 2+ , in contrast to the highly Ca 2+ selective concatenated Orai1 tetramer and native Orai1 channels [39] . Importantly, our STIM1 oligomerization model predicts that CC1 and CC2 mediate intradimer supercoiling essential to maintain the dimer unit building blocks of the STIM1-activation apparatus, while CC3 coordinates the assembly of these units to present a tetramer, hexamer or any other even-numbered multimeric structure to the cytoplasmic face of the Orai1 proteins for coupling and activation. 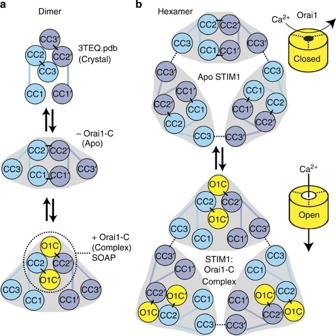Figure 5: Schematic of STIM1/Orai1 CC interplay in SOCE regulation. CC interactions in the assembly of dimers (a) and hexamers (b). The SOAP is indicated (broken black circle). STIM1 domains from individual subunits are cyan and light blue, while the Orai1 C-terminal domains are yellow. Sites of CC interactions are indicated (solid black lines). The assembly of STIM1 dimer units occurs through CC3:CC3′ interactions (broken black lines). Yellow cylinders represent the Orai1 channel with each dimer unit separated by a broken line. Channels are closed in the absence of STIM1 binding; however, interactions through CC1[TM-distal]-CC2:Orai1 C272–292supercoiling (elucidated herein) and via Orai1 N-terminal domain (currently unresolved) open the channel pore. CC1 refers to the CC1[TM-distal]region; CC1[TM-proximal]interactions known to have a vital role in the quiescent-to-active conformational switch32,38are not depicted. Figure 5: Schematic of STIM1/Orai1 CC interplay in SOCE regulation. CC interactions in the assembly of dimers ( a ) and hexamers ( b ). The SOAP is indicated (broken black circle). STIM1 domains from individual subunits are cyan and light blue, while the Orai1 C-terminal domains are yellow. Sites of CC interactions are indicated (solid black lines). The assembly of STIM1 dimer units occurs through CC3:CC3′ interactions (broken black lines). Yellow cylinders represent the Orai1 channel with each dimer unit separated by a broken line. Channels are closed in the absence of STIM1 binding; however, interactions through CC1 [TM-distal] -CC2:Orai1 C 272–292 supercoiling (elucidated herein) and via Orai1 N-terminal domain (currently unresolved) open the channel pore. CC1 refers to the CC1 [TM-distal] region; CC1 [TM-proximal] interactions known to have a vital role in the quiescent-to-active conformational switch [32] , [38] are not depicted. Full size image We suggest that the binding-induced arrangement of the Orai1 C-termini within each STIM1 dimer is a key step in eliciting an Orai1 subunit reorientation necessary for channel-gating. At ER–PM junctions, two Orai1 C-termini couple to the α2:α2′ SOAP formed by each STIM1 dimer, stabilized by CC2:Orai1 C 272–292 supercoiling ( Fig. 5a,b ; Supplementary Fig. S13a ). The D. melanogaster Orai C-terminal helices are inwardly twisted compared with the human Orai1 C 272–292 following structural alignment of the homologous residues ( Supplementary Fig. S13b ). Hence, we speculate that the interaction not only recruits Orai1 to the ER–PM junctions but also causes an allosteric movement in the Orai1 TM helices, an outward angular rotation of both TM4 helices, for example ( Supplementary Fig. S13b ), necessary for channel activation. A dual role for the Orai1 C-terminal domain in recruitment and gating is consistent with Orai1–CAD fusions that exhibit no channel activity when Orai1 residues 272–279 are deleted, despite forced colocalization [29] . It should be noted that the D. melanogaster Orai and human Orai1 sequence identity is only ~25% through the final 32 C-terminal residues ( Fig. 4c ) and, thus, the observed structural differences may partly originate from this incongruity. The Orai1 N-terminal residues 70/74–91 are also required for gating of the pore [18] , [19] and enhance trapping of channels at ER–PM junctions [29] . Considering that CC2–CC3 STIM1 fragments are the minimal activating regions within STIM1 (refs 18 , 19 , 20 ), Orai1 N-terminal interactions with CC2, CC3 or other regions of Orai1 must also occur for channel activity. Precise elucidation of the N-terminal-coupling mechanisms and allosteric conformational changes vital for Orai1 channel activation requires further structural work. Protein expression and purification The 6 × His-tagged STIM1 constructs (that is, residues 234–474/491 (OASF and OASF ext , respectively), residues 312–387 (renamed CC1 [TM-distal] -CC2); residues 388–491 (renamed CC3); a concatenated version of these regions including residues 312–491 (renamed CC1 [TM-distal] -CC2-CC3) ( Fig. 1a )) were cloned into pET-28a using the Nhe I/ Xho I sites. STIM proteins were expressed in BL21-ΔE3 Escherichia coli at 24 °C overnight and pulled out of crude lysate solubilized with 6 M guanidine HCl, 20 mM TRIS, 7.5 mM β-mercaptoethanol (BME), pH 8 using Ni-NTA agarose (Qiagen Inc.). Subsequently, the agarose resin was washed in 6 M urea, 20 mM TRIS, 1 mM dithiothreitol, pH 8, and protein was eluted using wash buffer supplemented with 350 mM imidazole. After dialysis (that is, 6,000–8,000 molecular weight cutoff; Spectra/Por membrane) and overnight digestion with bovine thrombin at 4 °C (12.5 units mg −1 protein), gel filtration chromatography (that is, Superdex S200 10/300 GL; GE Healthcare Inc.) in 20 mM TRIS, 300 mM NaCl, 1 mM DTT, pH 7.3 and 8 (that is, pH 8 for OASF, OASF ext and CC1 [TM-distal] -CC2-CC3; pH 7.3 for CC1 [TM-distal] -CC2) was employed as a final purification step. Protein homogeneity to >95% was confirmed with Coomassie blue-stained SDS–PAGE. The commercially available QuikChange kit (Stratagene Inc.) was used for the introduction of point mutations, and all mutagenesis was confirmed with the help of DNA sequencing (ACGT Corp.). The Orai1 C 272–292 fragment ( Fig. 1b ) cloned in pGEX-4T1 using the Bam HI/ Eco RI sites was expressed in BL21-ΔE3 E. coli at 37 °C for 4 h. Cell lysate was collected after resuspension in phosphate-buffered saline, probe-sonication on ice and incubation in the presence of 1% (v/v) Triton X100 and 2 mM BME at 4 °C. The GST fusions were pulled out of the lysate using GST Sepharose 4B beads (GE Healthcare Inc.), washed with phosphate-buffered saline in the presence of 2 mM BME and eluted with 20 mM TRIS, 150 mM NaCl, 2 mM DTT and 10 mM reduced glutathione, pH 7.5. Subsequently, the GST was cleaved by overnight incubation with bovine thrombin (that is, 15 units mg −1 fusion protein, 20 mM TRIS, 150 mM NaCl, pH 7.5, 4 °C). Free Orai1 C 272–292 was collected and concentrated using ultrafiltration, sequentially through 10,000 Da and 2,000 Da molecular weight cutoff membranes. The mass of intact Orai1 C 272–292 was confirmed using mass spectrometry. The Orai1 C 272–292 fragment was cloned into a pMAL-c2x vector using Bam HI/ Eco RI sites and expressed in BL21-ΔE3 E. coli at 15 °C overnight. Cells were lysed after resuspension in 20 mM TRIS, 200 mM NaCl, 1 mM EDTA, pH 7.5 using probe-sonication on ice, and after incubation at 4 °C in the presence of 0.1% (v/v) Triton X100 and 2 mM BME, the MBP fusions were pulled out of the lysate using Amylose resin (New England Biolabs Inc.). Subsequently, the resin was washed in 20 mM TRIS, 200 mM NaCl, 1 mM EDTA, 0.1% (v/v) Triton X100, 2 mM BME, pH 7.5, and the protein was eluted with wash buffer supplemented with 10 mM maltose. Unless otherwise stated, the buffer was 20 mM TRIS, 300 mM NaCl, 2 mM DTT, pH 7.3 for all in vitro experiments involving recombinant proteins. Solution NMR spectroscopy NMR experiments were performed on 600 and 800 MHz Avance (Bruker Biospin Ltd.) spectrometers equipped with cryogenic, triple-resonance probes (1.7 and 5 mm, respectively). Unless otherwise stated, the NMR buffer was 20 mM bisTRIS and 17.5% (v/v) TFE, pH 5.5. Backbone data were acquired using standard 1 H- 15 N-HSQC, 1 H- 15 N- 13 C-HNCO [40] , CBCA(CO)NH [41] and HNCACB [42] experiments, while side-chain data were obtained using 1 H- 13 C-HSQC, H(C)(CO)NH-TOCSY [43] and (H)C(CO)NH-TOCSY [43] , [44] experiments. NOE data from 15 N-edited and 13 C-edited 3D NOESY-HSQC (three-dimensional nuclear Överhauser enhancement spectroscopy-HSQC) experiments also aided in the assignments [45] . 15 N relaxation data were acquired in the presence and absence of a 3-s 1 H saturation period before 15 N excitation using the 15 N-{ 1 H} heteronuclear NOE pulse sequence [46] . All spectra were processed using NMRPipe [47] , and chemical shifts were assigned using XEASY [48] . NMR structure calculations Dihedral angle restraints were calculated from chemical shifts using TALOS [49] . Hydrogen bond restraints were inferred from the chemical-shift index [50] and TALOS secondary structure output. CYANA (v3.0) was used for automated NOE assignment and structure calculation based on >92% complete chemical-shift assignments and 3D NOESY-HSQC peak lists using default dimer symmetry weighting [51] , [52] . For the apo CC1 [TM-distal] -CC2 calculation, 13 C/ 15 N-filtered/ 13 C-edited [53] , [54] , 13 C/ 15 N-filtered/ 15 N-edited [53] , [54] , 15 N-edited and 13 C-edited NOESY [45] spectra were used for distance-restraint derivation, using 1:1 mixtures of 15 N- 13 C-labelled and -unlabelled protein (~1.2 mM total protein). Distance restraints for the CC1 [TM-distal] -CC2:Orai1 C 272–292 complex were derived from 15 N-edited- and 13 C-edited NOESY [45] spectra of mixtures of 15 N- 13 C-labelled CC1 [TM-distal] -CC2 (~0.25 mM) with unlabelled Orai1 C 272–292 (~2.5 mM), and 15 N- 13 C-labelled Orai1 C 272–292 (~0.4 mM) with unlabelled CC1 [TM-distal] -CC2 (~3.0 mM). The lack of filtered restraints for the complex because of the relatively weak Orai1 C 272–292 -binding affinity was compensated by the high-level chemical-shift assignments (that is, >92%) in the structure calculation using non-distinctive inter- and intramolecular NOESY data [51] . Water-refinement and violation analysis was performed using the RECOORD scripts [55] in CNS (v1.1) [56] . Structure quality (that is, Ramachandran statistics) was assessed using PROCHECK-NMR [57] . No constraints were derived from the D. melanogaster Orai crystal structure (4HKR.pdb). Structure images were rendered in PyMOL [58] . STIM1 subunits are distinguished by cyan and light blue colouring, Orai1 C 272–292 helices are coloured yellow, N and C denote amino and carboxy termini, respectively, and side-chain positions are shown for the lowest energy 20 structure ensemble. Solution small angle X-ray and DLS To verify that the overall conformation of CC1 [TM-distal] -CC2 is not influenced by TFE, we collected solution SAXS and DLS data. X-Ray scattering measurements were carried out at the 12-ID-C beamline of the Advanced Photon Source, Argonne National Laboratory (Argonne, IL). The energy of the X-ray beam was 18 keV (wavelength, λ =0.6888 Å). The sample to charge-coupled device detector (MAR research, Hamburg) distances were adjusted to achieve scattering q values of 0.006<q<0.28 Å −1 , where q =(4 π / λ )sin θ , and 2 θ is the scattering angle. Twenty two-dimensional images were recorded for each buffer or sample using a flow cell at 4 °C, with an accumulated exposure time of 1–2 s to reduce radiation damage. No radiation damage was observed as confirmed by the absence of systematic signal changes in sequentially collected X-ray scattering images. DLS measurements were made on a temperature-controlled Dynapro Titan (Wyatt Technology) using a 12 μl, 8.5 mm centre height quartz cuvette. The incident laser light was 827.4 nm, the scattering angle was 90° and the temperature was 20 °C. Analysis was performed using the accompanying Dynamics software version 6.7.7.9 (Wyatt Technology). Solution NMR-binding assays Equilibrium dissociation constants ( K d ) were calculated from plots of chemical-shift perturbation versus CC1 [TM-distal] -CC2 concentration in monomers. All 1 H- 15 N-HSQC titration spectra were referenced by overlaying the H(N) resonance of free 15 N -acetyl-Gly. The NMRPipe titration analysis scripts were used to evaluate the NMR-binding curves separately based on 15 N- and 1 H- Orai1 C 272–292 chemical-shift changes as a function of unlabelled CC1 [TM-distal] -CC2 concentration, and the binding data were fit to a one-site binding model per monomer (that is, two sites per dimer) [47] . The model recapitulated the perturbation curves well, and the extracted K d values ranged from ~100 to 600 μM, depending on the resonance and sample analysed ( Supplementary Fig. S7e ). The presence of TFE prohibits the direct translation of the K d values to a physiological context because of the weakening affects of the co-solvent on protein interactions ( Supplementary Discussion ); however, we used a conservative K d =400 μM to simulate the concentration of peptide required to saturate >85% of a 400 μM solution of STIM1 CC1 [TM-distal] -CC2 (that is, ~3 mM peptide) and prepared our NMR samples for structure determination of the complex accordingly. MBP pull-down binding assays MBP-Orai1 C 272–292 (that is, 25 μl of 10 μM) was incubated with buffer-equilibrated amylose resin (that is, 25 μl) for 15 min at ambient temperature. After excess solution was removed using centrifugation, CC1 [TM-distal] -CC2 (that is, 75 μl of 50 μM) was added to the resin and incubated for 10 min. The resin was washed with buffer (3 × 750 μl) and water (2 × 1,000 μl), removing the solution using centrifugation at each step. The resin was boiled in 1 × SDS–PAGE loading dye (that is, 80 μl) for 5 min and supernatants were separated on 12.5% SDS–PAGE gels. All centrifugation steps were at 16,000 g for 1 min and 4 °C. SEC with in-line light scattering SEC was performed on Superdex S200 10/300 GL columns by using an AKTA FPLC system (GE Healthcare Life Sciences) at 4 °C. MALS measurements were carried out in-line with SEC by using a three-angle (45°, 90° and 135°) miniDawn light-scattering instrument equipped with a 690 nm laser and an Optilab rEX differential refractometer (Wyatt Technologies Inc.). Molecular weight was calculated by using the ASTRA software (Wyatt Technologies Inc.) based on the Zimm plot analysis and by using a protein refractive index increment, dn dc −1 =0.185 L g −1 . Circular dichroism Data were acquired on a Jasco J-815 CD Spectrometer (Jasco Inc.) in 1 nm increments (20 nm min −1 ) by using 0.1 cm pathlength cuvettes, an 8-s averaging time and 1 nm bandwidth. Spectra were corrected for buffer contributions. Thermal melts were acquired by monitoring the change in the 222-nm CD signal as a function of temperature in 0.1 cm cuvettes, an 8-s averaging time, 1 nm bandwidth and a 1 °C min −1 scan rate. Whole-cell HEK-293 patch-clamp experiments HEK-293 cells (DSMZ, Braunschweig, Germany) were transfected (Transfectin, Bio-Rad) with 1 μg DNA of YFP-Orai1 and mCh-STIM1 constructs. Electrophysiological experiments were performed after 24–34 h, using the patch-clamp technique in whole-cell recording configurations at 21–25 °C. Cells were selected for analyses based on similar cell-to-cell mCh-STIM1 as well as cell-to-cell YFP-Orai1 expression levels by fluorescence intensity. The fluorescence intensity of mCh-STIM1 and YFP-Orai1 partially active mutants did not exhibit significantly altered expression levels compared with the wild-type proteins when transfected under similar conditions. An Ag/AgCl electrode was used as the reference electrode. Voltage ramps were applied every 5 s from a holding potential of 0 mV, covering a range of −90 to 90 mV over 1 s. For passive store depletion, the internal pipette solution included (in mM) the following: 145 Cs methane sulphonate, 20 EGTA, 10 HEPES, 8 NaCl, 3.5 MgCl 2 and pH 7.2. Standard extracellular solution consisted of (in mM) 145 NaCl, 10 HEPES, 10 CaCl 2 , 10 glucose, 5 CsCl, 1 MgCl 2 and pH 7.4. A liquid junction potential correction of +12 mV was applied, resulting from a Cl − -based bath solution and a sulphonate-based pipette solution. All currents were leak-subtracted either by subtracting the initial voltage ramps obtained shortly following break-in with no visible current activation, or with constitutively active currents after 10 μM La 3+ application at the end of the experiment. In STIM1/Orai1 co-overexpressing HEK-293 cells, no other currents besides CRAC currents by store depletion are stimulated and the currents display classic CRAC channel biophysical characteristics; hence, La 3+ can be reliably used to inhibit Orai1 currents, shown only for constitutively active CRAC current traces. Accession codes: The structure coordinates are deposited in the RCSB protein data bank (pdb codes: 2MAJ.pdb and 2MAK.pdb). NMR chemical shifts and structure constraints are deposited in the BMRB (accession codes: 19362 and 19363). How to cite this article: Stathopulos, P. B. et al. STIM1/Orai1 coiled-coil interplay in the regulation of store-operated calcium entry. Nat. Commun. 4:2963 doi: 10.1038/ncomms3963 (2013).